The epigenetic modifier EZH2 controls melanoma growth and metastasis through silencing of distinct tumour suppressors Increased activity of the epigenetic modifier EZH2 has been associated with different cancers. However, evidence for a functional role of EZH2 in tumorigenesis in vivo remains poor, in particular in metastasizing solid cancers. Here we reveal central roles of EZH2 in promoting growth and metastasis of cutaneous melanoma. In a melanoma mouse model, conditional Ezh2 ablation as much as treatment with the preclinical EZH2 inhibitor GSK503 stabilizes the disease through inhibition of growth and virtually abolishes metastases formation without affecting normal melanocyte biology. Comparably, in human melanoma cells, EZH2 inactivation impairs proliferation and invasiveness, accompanied by re-expression of tumour suppressors connected to increased patient survival. These EZH2 target genes suppress either melanoma growth or metastasis in vivo , revealing the dual function of EZH2 in promoting tumour progression. Thus, EZH2-mediated epigenetic repression is highly relevant especially during advanced melanoma progression, which makes EZH2 a promising target for novel melanoma therapies. Melanoma is the most deadly skin cancer, with a yearly increasing incidence rate [1] . Its aggressiveness is based on the highly metastatic potential of melanoma cells, which can still not be efficiently targeted despite recent progress in melanoma therapies [2] . In fact, currently available drugs frequently induce resistance [3] and have even been shown to promote invasiveness and metastasis of resistant cells [4] . Thus, new treatments for metastatic melanoma need to be established. Melanoma arises from melanocytes that originate during embryonic development from neural crest stem cells (NCSCs) [5] . In the embryo, neural crest cells delaminate from the neural tube by undergoing an epithelial-to-mesenchymal transition (EMT) [6] , a process also implicated in early steps of tumour metastasis [7] . Upon EMT, neural crest cells adopt stem cell features and a remarkable migratory capacity, which allows the cells to disseminate through the embryonic tissue and to colonize distant sites, including the skin where they give rise to melanocytes [8] . Tumorigenesis from these cells is induced by acquired driver mutations, for instance in the NRAS or BRAF locus [9] , [10] . Moreover, genes known to regulate NCSCs and melanocyte development have been associated with melanoma formation. For instance, the small Rho GTPase Rac1 controls self-renewal and expansion of post migratory NCSCs [11] , and activating mutations in RAC1 drive melanoma formation [9] , [10] . Likewise, the transcription factor Sox10 promotes both NCSC maintenance and melanomagenesis in a murine melanoma model [12] , [13] , [14] . Apart from genetic factors, aberrant epigenetic control also frequently leads to developmental disorders [15] and has been connected to oncogenesis [16] . A prominent epigenetic modifier is enhancer of zeste homologue 2 (EZH2), which is a component of the polycomb repressive complex 2. EZH2 contains a SET domain, the catalytic subunit of histone methyltransferases, which catalyses trimethylation of lysine 27 in histone 3 (H3K27me3), and thus induces chromatin compaction and consequently prevents transcription of target genes [17] , [18] . During embryonic development and in tissue-specific stem cells, EZH2-mediated transcriptional repression often targets lineage commitment or differentiation [17] , [19] , [20] . Therefore, in many systems, EZH2 activity supports stem cell maintenance by repressing differentiation. In contrast, in NCSCs Ezh2 neither represses differentiation nor controls stem cell proliferation, but rather promotes the acquisition of a mesenchymal fate [21] . In a wide variety of cancers including melanoma, EZH2 expression is elevated and associated with poor survival [22] , [23] , [24] . In cancer, EZH2 function has predominantly been associated with proliferation and tumour growth, comparable to its role in embryonic and adult tissues [22] . Most of these data have been gathered by means of in vitro culture and tumour cell xenograft assays, while studies on the role of EZH2 in physiological in vivo models of tumorigenesis are sparse and only focus on hyperplastic transformation of normal cells rather than progression into metastatic disease [25] , [26] , [27] . In human melanoma cells, loss of EZH2 partially interfered with proliferation or invasion capacity, dependent on the cell line and the experimental set up used [28] , [29] , [30] . However, a study investigating EZH2 function in a physiological context of melanoma progression, from tumour initiation to metastatic disease, is still missing. In the present work, we identify essential roles of EZH2 for the initiation and progression of metastatic melanoma in vivo and reveal novel tumour suppressors regulated by EZH2. These tumour suppressors represent two distinct sets of target genes that are either involved in regulating proliferation or metastasis formation. Therefore, blocking EZH2 activity might represent a powerful strategy for the development of novel therapies interfering with distinct aspects of melanomagenesis. EZH2 is highly expressed in human and murine melanoma Previously, high EZH2 expression has been described in biopsies of malignant melanoma in comparison to benign naevi [23] , [24] . To address whether changes in EZH2 expression affect cells of the melanocytic lineage rather than stromal cells in the tumour tissue, we performed co-staining of human cutaneous melanoma sections for EZH2 in combination with SOX10 or MART1-HMB45, all markers for the melanocytic lineage [14] , [31] , [32] , [33] . In agreement with previous studies [23] , [24] , human primary melanomas and metastases displayed high EZH2 expression in cells of the melanocytic lineage compared with epidermal melanocytes and dermal naevus cells ( Fig. 1a ; Supplementary Fig. 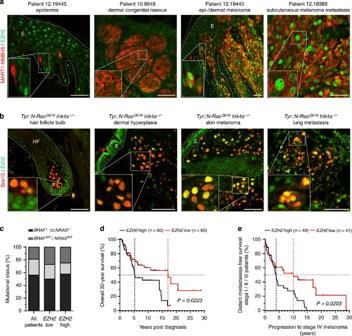Figure 1: EZH2 is upregulated in melanoma and correlates with adverse patient survival. (a) Immunofluorescent staining for HMB45-MART1 and EZH2 on human epidermis, congenital naevus, primary melanoma and subcutaneous melanoma metastasis sections from biopsies described in (Supplementary Table 1). (b) Immunofluorescent staining for Sox10 and Ezh2 on skin and lung sections of melanoma-developingTyr::N-RasQ61KInk4a−/−mice. (c)BRAFandNRASmutational status of melanoma specimens included inEZH2TCGA analysis. All patients,n=274;EZH2low,n=60;EZH2high,n=60. (d) Kaplan–Meier curves comparing overall survival of melanoma specimens (stage I–IV) with respect toEZH2transcript levels based on TCGA. (e) Kaplan–Meier curves comparing distant metastases-free survival of stage I–III melanoma specimens (primary melanoma/lymph node metastases) with respect toEZH2transcript levels based on TCGA. E, epidermis;EZH2low/high, bottom and top 60 patients with respect toEZH2transcript levels; HF, hair follicle.Pvalues calculated with log-rank (Mantel–Cox) test. Scale bars, 50 μm. 1 ; Supplementary Table 1 ). To study the function of Ezh2 in an in vivo context of melanoma development, we took advantage of a mouse model of cutaneous melanoma. Tyr::N-Ras Q61K Ink4a −/− mice display dermal hyperplasia reminiscent of human congenital naevi and consistently develop metastatic melanoma within 6 months of age [14] , [34] . Similar to human patients, Ezh2 protein was strongly expressed in Sox10-positive cells of murine skin melanoma and distant metastases. In contrast, Sox10-expressing cells in hair follicle bulbs, the physiological location of melanocytes in murine trunk skin [35] , and in dermal hyperplasia only showed marginal Ezh2 expression ( Fig. 1b ), consistent with the human data. Figure 1: EZH2 is upregulated in melanoma and correlates with adverse patient survival. ( a ) Immunofluorescent staining for HMB45-MART1 and EZH2 on human epidermis, congenital naevus, primary melanoma and subcutaneous melanoma metastasis sections from biopsies described in ( Supplementary Table 1 ). ( b ) Immunofluorescent staining for Sox10 and Ezh2 on skin and lung sections of melanoma-developing Tyr::N-Ras Q61K Ink4a −/− mice. ( c ) BRAF and NRAS mutational status of melanoma specimens included in EZH2 TCGA analysis. All patients, n =274; EZH2 low, n =60; EZH2 high, n =60. ( d ) Kaplan–Meier curves comparing overall survival of melanoma specimens (stage I–IV) with respect to EZH2 transcript levels based on TCGA. ( e ) Kaplan–Meier curves comparing distant metastases-free survival of stage I–III melanoma specimens (primary melanoma/lymph node metastases) with respect to EZH2 transcript levels based on TCGA. E, epidermis; EZH2 low/high, bottom and top 60 patients with respect to EZH2 transcript levels; HF, hair follicle. P values calculated with log-rank (Mantel–Cox) test. Scale bars, 50 μm. Full size image Increased EZH2 expression is linked to poor patient survival To study the significance of high EZH2 expression for the survival of cutaneous melanoma patients, we established an EZH2 high and an EZH2 low patient group based on RNAseq and clinical data from The Cancer Genome Atlas (TCGA). These groups did not display obvious differences with respect to clinically relevant factors including BRAF and NRAS mutations ( Fig. 1c ). However, patients of the EZH2 high group showed a significantly shorter overall survival as compared with those of the EZH2 low group ( Fig. 1d ). Intriguingly, primary melanoma and lymph node metastases patients (stage I–III) of the EZH2 high group developed distant metastases (stage IV) significantly faster than EZH2 low-expressing stage I–III patients ( Fig. 1e ), implying a potential role of EZH2 in metastatic spread of melanoma. Apart from expression levels, mutations affecting EZH2 activity have been implicated in malignancies, predominantly of the haematopoietic system [36] . We analyzed the occurrence of EZH2 somatic mutations in cutaneous melanoma in comparison to nine different cancer types using TCGA and four further data sets [9] , [10] , [37] , [38] . In this analysis, cutaneous melanoma showed the highest non-synonymous EZH2 mutation frequency besides primary lymphomas (including follicular and diffuse large B-cell lymphomas). In particular, cutaneous melanoma was the only solid cancer with non-synonymous mutations affecting tyrosine 646 (Y646*) in the SET domain of EZH2 ( Fig. 2a,b ) (EZH2 Y646* based on current NCBI protein reference sequence NP_004447.2; earlier referred as EZH2 Y641* based on NP_001190176.1). Previously, EZH2 Y646* mutations were reported to be widely present in primary lymphoma and to lead to increased EZH2 activity resulting in aberrant H3K27me3 (ref. 36 ). To associate EZH2 non-synonymous mutations present in melanoma patients with EZH2 function, we overexpressed selected EZH2 mutations in vitro . However, except EZH2 Y646* , none of the mutations analyzed induced an increase in global H3K27me3 ( Fig. 2c,d ). Further functional studies are necessary to uncover properties of these mutations that might allow a functional link to cutaneous melanomagenesis. 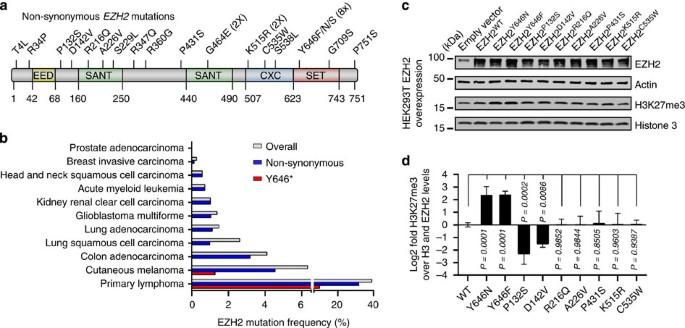Figure 2:EZH2is frequently mutated in human melanoma. (a)EZH2non-synonymous mutational landscape includingEZH2Y646*-activating mutations based on TCGA melanoma data set and three further data sets9,10,37. (b)EZH2mutation frequencies including Y646* in different cancers based on TCGA and two further data sets9,38. (c,d) Western blot for EZH2 protein and H3K27me3 on HEK293T cells overexpressing differentEZH2mutations to quantify changes in H3K27me3. WT, wild type. Data are represented as mean±s.e.m. ofn=4.Pvalues calculated with analysis of variance and Fisher’s least significant difference test. Figure 2: EZH2 is frequently mutated in human melanoma. ( a ) EZH2 non-synonymous mutational landscape including EZH2 Y646* -activating mutations based on TCGA melanoma data set and three further data sets [9] , [10] , [37] . ( b ) EZH2 mutation frequencies including Y646* in different cancers based on TCGA and two further data sets [9] , [38] . ( c , d ) Western blot for EZH2 protein and H3K27me3 on HEK293T cells overexpressing different EZH2 mutations to quantify changes in H3K27me3. WT, wild type. Data are represented as mean±s.e.m. of n =4. P values calculated with analysis of variance and Fisher’s least significant difference test. Full size image Ezh2 function is dispensable for homeostasis of melanocytes Because EZH2 was highly expressed in human and murine melanoma and linked to poor patient survival, we studied its function in vivo. To this end, mice carrying floxed alleles of the Ezh2 locus [19] were used to conditionally delete Ezh2 in the melanocytic lineage by tamoxifen (TM)-induced activation of Cre-recombinase ( Tyr::Cre ERT2 ) [39] . Inclusion of a Cre-reporter allele ( R26R::LacZ ) [40] allowed fate mapping of recombined cells in vivo . To address a potential role of Ezh2 in maintaining normal melanocytic function, Ezh2 was conditionally depleted in tumour-free Tyr::Cre ERT2 Ezh2 lox/lox R26R::LacZ mice ( Fig. 3a ). TM was applied to 1-month-old animals, and mice were monitored for hair greying ( Fig. 3b ). Hair greying is the phenotype predominantly arising upon interference with homeostasis of melanocyte stem cells in the bulge [31] , [41] , the permanent niche of epithelial and melanocyte stem cells in hair follicles [35] , [42] . However, hair pigmentation remained normal up to 1 year after Ezh2 depletion ( Fig. 3c ). Importantly, Ezh2 was efficiently and durably ablated in melanocytes of trunk skin hair follicles, leading to a concomitant loss of H3K27me3 ( Fig. 3d,e ). 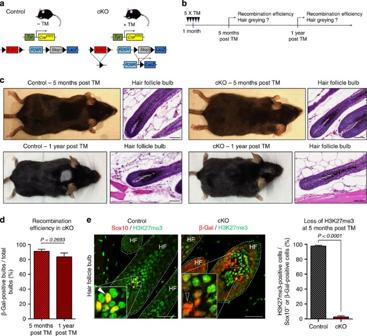Figure 3: Ezh2 is not required for normal melanocyte homeostasis. (a,b) Mouse genotypes (a) and strategy (b) used to analyze the effect of conditionalEzh2ablation in the melanocytic lineage of adult wild type mice. (c) Macroscopic pictures and H&E staining on trunk skin sections of control and cKO mice at 5 months and 1 year post conditionalEzh2ablation. (d) Immunofluorescent staining on trunk skin sections of wt mice for β-Gal to quantify recombination efficiencies (representative fields not shown). (e) Immunofluorescent staining on trunk skin sections of wt mice for Sox10 (control) or β-Gal (cKO) and H3K27me3 to quantify H3K27me3 depletion. White arrowhead, Sox10-positive cell considered H3K27me3 positive; white open arrowhead, β-Gal-positive cell considered H3K27me3 negative. H&E, haematoxylin and eosin; HF, hair follicle. Data are represented as mean±s.e.m. ofn=3.Pvalues calculated with unpaired Student’st-test. Scale bars, 50 μm. Figure 3: Ezh2 is not required for normal melanocyte homeostasis. ( a , b ) Mouse genotypes ( a ) and strategy ( b ) used to analyze the effect of conditional Ezh2 ablation in the melanocytic lineage of adult wild type mice. ( c ) Macroscopic pictures and H&E staining on trunk skin sections of control and cKO mice at 5 months and 1 year post conditional Ezh2 ablation. ( d ) Immunofluorescent staining on trunk skin sections of wt mice for β-Gal to quantify recombination efficiencies (representative fields not shown). ( e ) Immunofluorescent staining on trunk skin sections of wt mice for Sox10 (control) or β-Gal (cKO) and H3K27me3 to quantify H3K27me3 depletion. White arrowhead, Sox10-positive cell considered H3K27me3 positive; white open arrowhead, β-Gal-positive cell considered H3K27me3 negative. H&E, haematoxylin and eosin; HF, hair follicle. Data are represented as mean±s.e.m. of n =3. P values calculated with unpaired Student’s t -test. Scale bars, 50 μm. Full size image N-Ras Q61K -expressing naevus cells are Ezh2 independent This unforeseen independence of the normal melanocyte lineage from Ezh2-mediated gene repression prompted us to investigate a possible function of Ezh2 in maintaining benign naevus-like dermal hyperplasia. Therefore, Ezh2 was depleted in our genetic Tyr::N-Ras Q61K Ink4a −/− Tyr::Cre ERT2 Ezh2 lox/lox R26R::LacZ melanoma model ( Fig. 4a,b ; Supplementary Fig. 2a–c ). As in tumour-free mice, conditional deletion of Ezh2 in Tyr::N-Ras Q61K Ink4a −/− animals had no effect on hair pigmentation ( Fig. 4c ; Supplementary Fig. 2d ). Importantly, maintenance of benign dermal hyperplasia was also not affected ( Supplementary Fig. 2d ), despite efficient Ezh2 depletion and subsequent loss of H3K27me3 ( Supplementary Fig. 2e,f ). Even when aged for up to 1 year after conditional knockout (cKO) of Ezh2 , Tyr::N-Ras Q61K mice with functional Ink4a wt (wild type) loci did not show an overt reduction of recombined melanocytic cells in the dermis ( Supplementary Fig. 2e ). Accordingly, dermal hyperplasia grew to a similar size with a comparably low proliferation rate in both control and Ezh2 -depleted mice ( Fig. 4d,e ). Thus, Ezh2-mediated gene repression is dispensable for both physiological homeostasis of normal melanocytes and maintenance of N-Ras Q61K -transformed cells in dermal hyperplasia, independent of Ink4a -deficiency. 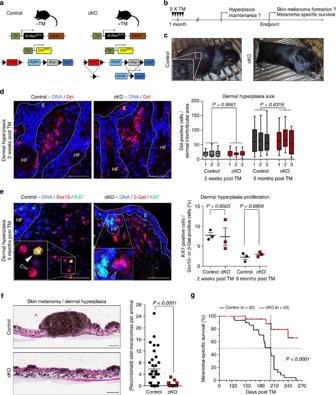Figure 4:Ezh2ablation inTyr::N-RasQ61KInk4a−/−mice prevents skin melanoma formation. (a,b) Mouse genotypes (a) and strategy (b) used to analyze the effect of conditionalEzh2ablation on dermal hyperplasia and melanoma formation inTyr::N-RasQ61KInk4a−/−mice. (c) Macroscopic pictures of a control and a cKO littermate at 5 months postEzh2ablation. (d) Immunofluorescent staining for Dct on trunk skin sections 2 weeks after conditionalEzh2ablation to quantify dermal hyperplasia size. (e) Immunofluorescent staining for Sox10 (control) or β-Gal (cKO) and Ki67 on trunk skin sections 5 months after conditionalEzh2ablation to quantify proliferation rates. White arrowhead, Sox10-positive/Ki67-positive cell; white open arrowheads, Sox10- or β-Gal-positive/Ki67-negative cells. (f) H&E staining on trunk skin sections of control and cKO mice at day of sacrifice to quantify skin melanoma numbers. (g) Kaplan–Meier curves comparing melanoma-specific survival after conditionalEzh2ablation. For cKO mice, only recombined skin melanomas were taken into count as in (Supplementary Fig. 3e). E, epidermis; HF, hair follicle; H&E, haematoxylin and eosin. Data are represented as median±100% range ofn≥20 interfollicular areas, three animals per group (d), mean±s.e.m. ofn=3 (e), mean±s.e.m. ofn=32 (control),n=23 (cKO) (f).Pvalues calculated with unpaired Student’st-test (d–f), log-rank (Mantel–Cox) test (g). Scale bars, 50 μm (d,e), 500 μm (f). Figure 4: Ezh2 ablation in Tyr::N-Ras Q61K Ink4a −/− mice prevents skin melanoma formation. ( a , b ) Mouse genotypes ( a ) and strategy ( b ) used to analyze the effect of conditional Ezh2 ablation on dermal hyperplasia and melanoma formation in Tyr::N-Ras Q61K Ink4a −/− mice. ( c ) Macroscopic pictures of a control and a cKO littermate at 5 months post Ezh2 ablation. ( d ) Immunofluorescent staining for Dct on trunk skin sections 2 weeks after conditional Ezh2 ablation to quantify dermal hyperplasia size. ( e ) Immunofluorescent staining for Sox10 (control) or β-Gal (cKO) and Ki67 on trunk skin sections 5 months after conditional Ezh2 ablation to quantify proliferation rates. White arrowhead, Sox10-positive/Ki67-positive cell; white open arrowheads, Sox10- or β-Gal-positive/Ki67-negative cells. ( f ) H&E staining on trunk skin sections of control and cKO mice at day of sacrifice to quantify skin melanoma numbers. ( g ) Kaplan–Meier curves comparing melanoma-specific survival after conditional Ezh2 ablation. For cKO mice, only recombined skin melanomas were taken into count as in ( Supplementary Fig. 3e ). E, epidermis; HF, hair follicle; H&E, haematoxylin and eosin. Data are represented as median±100% range of n ≥20 interfollicular areas, three animals per group ( d ), mean±s.e.m. of n =3 ( e ), mean±s.e.m. of n =32 (control), n =23 (cKO) ( f ). P values calculated with unpaired Student’s t -test ( d – f ), log-rank (Mantel–Cox) test ( g ). Scale bars, 50 μm ( d , e ), 500 μm ( f ). Full size image Ezh2 function is essential for melanoma initiation To assess a possible role of Ezh2 in tumorigenesis, Ezh2 was conditionally deleted in our murine melanoma model before appearance of cutaneous tumours ( Fig. 4a,b ; Supplementary Fig. 3a,b ). While in control mice, many skin melanomas (Ø≥2 mm) emerged after ~5 months, appearance of tumours was delayed in Ezh2 cKO animals ( Fig. 4c ; Supplementary Fig. 3c ) leading to an increased skin melanoma-free survival ( Supplementary Fig. 3d ). At day of sacrifice, the number of recombined skin melanomas was drastically reduced in Ezh2 cKO mice compared with the total tumour load in controls ( Fig. 4f ; Supplementary Fig. 3e ). In accordance with these data, melanoma-specific survival was significantly increased ( Fig. 4g ), independently of control type and sex of Ezh2 cKO mice ( Supplementary Fig. 3f ). Next, we addressed whether Ezh2 might also be implicated in melanoma progression after the onset of the disease. To this end, Tyr::N-Ras Q61K Ink4a −/− Tyr::Cre ERT2 Ezh2 lox/lox R26R::LacZ mice were individually monitored until appearance of skin melanomas ( Fig. 5d ; Supplementary Fig. 4f ). Ezh2 deletion was then induced by TM application ( Fig. 5a,b ; Supplementary Fig. 4a ). High recombination efficiency became apparent 1 month post TM application ( Supplementary Fig. 4b,c ). Concomitantly, this also led to an efficient loss of Ezh2 protein and H3K27me3 in recombined tumour cells ( Fig. 5c ; Supplementary Fig. 4d,e ). Frequent assessment of the animals showed a marked increase of new melanomas per week in control animals. In striking contrast, the tumour load was stabilized in Ezh2 cKO mice, in which virtually no new skin melanomas were emerging ( Fig. 5d ; Supplementary Fig. 4f ). Thus, early genetic interference with Ezh2 activity prevents progression of benign dermal hyperplasia into malignant cutaneous melanoma, while Ezh2 depletion in established melanoma effectively stops emergence of further skin tumours. 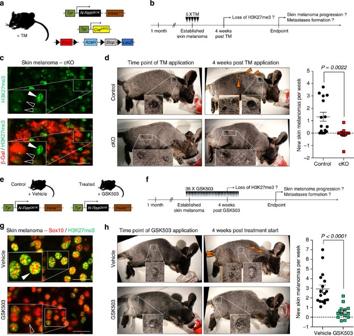Figure 5: Ezh2 inactivation in melanoma-bearing mice stabilizes the disease. (a,b) Mouse genotypes (a) and strategy (b) used to analyze the effect of conditionalEzh2ablation on melanoma progression inTyr::N-RasQ61KInk4a−/−mice. (c) Immunofluorescent staining for β-Gal and H3K27me3 on skin melanoma sections 4 weeks after conditionalEzh2ablation. White arrowhead, β-Gal-negative/H3K27me3-positive cell; white open arrowheads, β-Gal-positive/H3K27me3-negative cells. (d) Representative pictures ofTyr::N-RasQ61KInk4a−/−mice at time point ofEzh2ablation and 4 weeks later to quantify formation of new skin melanomas per week. Orange arrowheads, new skin melanomas. (e,f) Mouse genotypes (e) and strategy (f) used to analyze the effect of temporary GSK503 treatment onTyr::N-RasQ61KInk4a−/−mice with established melanoma. (g) Immunofluorescent staining on skin melanoma sections for Sox10 and H3K27me3 4 weeks after treatment start with vehicle or GSK503. White arrowhead, Sox10-positive/H3K27me3-positive cell; white open arrowhead, Sox10-positive/H3K27me3-negative cell. (h) Representative pictures ofTyr::N-RasQ61KInk4a−/−mice treated with vehicle or GSK503 at time point of treatment start and 4 weeks later to quantify formation of new skin melanomas per week. Orange arrowheads, new skin melanomas. H&E, haematoxylin and eosin. Data are represented as mean±s.e.m. ofn=15 (control)n=13 (cKO) (d), mean±s.e.m. ofn=17 (vehicle)n=15 (GSK503) (h).Pvalues calculated with unpaired Student’st-test. Scale bars, 25 μm. Figure 5: Ezh2 inactivation in melanoma-bearing mice stabilizes the disease. ( a , b ) Mouse genotypes ( a ) and strategy ( b ) used to analyze the effect of conditional Ezh2 ablation on melanoma progression in Tyr::N-Ras Q61K Ink4a −/− mice. ( c ) Immunofluorescent staining for β-Gal and H3K27me3 on skin melanoma sections 4 weeks after conditional Ezh2 ablation. White arrowhead, β-Gal-negative/H3K27me3-positive cell; white open arrowheads, β-Gal-positive/H3K27me3-negative cells. ( d ) Representative pictures of Tyr::N-Ras Q61K Ink4a −/− mice at time point of Ezh2 ablation and 4 weeks later to quantify formation of new skin melanomas per week. Orange arrowheads, new skin melanomas. ( e , f ) Mouse genotypes ( e ) and strategy ( f ) used to analyze the effect of temporary GSK503 treatment on Tyr::N-Ras Q61K Ink4a −/− mice with established melanoma. ( g ) Immunofluorescent staining on skin melanoma sections for Sox10 and H3K27me3 4 weeks after treatment start with vehicle or GSK503. White arrowhead, Sox10-positive/H3K27me3-positive cell; white open arrowhead, Sox10-positive/H3K27me3-negative cell. ( h ) Representative pictures of Tyr::N-Ras Q61K Ink4a −/− mice treated with vehicle or GSK503 at time point of treatment start and 4 weeks later to quantify formation of new skin melanomas per week. Orange arrowheads, new skin melanomas. H&E, haematoxylin and eosin. Data are represented as mean±s.e.m. of n =15 (control) n =13 (cKO) ( d ), mean±s.e.m. of n =17 (vehicle) n =15 (GSK503) ( h ). P values calculated with unpaired Student’s t -test. Scale bars, 25 μm. Full size image Ezh2-targeted therapy interferes with melanoma progression Our findings indicate that interference with EZH2 activity might be a valid strategy for therapy of advanced melanoma. To test this hypothesis, we treated mice with the preclinical EZH2 inhibitor GSK503, a small chemically optimized compound highly selective for the SET domain of EZH2 and exhibiting favourable pharmacokinetics in mice [27] . Independent of the genotype (wild type, Ink4a −/− or Tyr::N-Ras Q61K Ink4a −/− ), mice suffered from a tolerable and reversible weight loss of ~10% and, in rare cases, from development of ascites after prolonged treatment with GSK503. To investigate the effect of pharmacological Ezh2 inhibition on tumour progression, Tyr::N-Ras Q61K Ink4a −/− mice were individually monitored until skin melanomas were detectable ( Fig. 5h ; Supplementary Fig. 5c ) and subsequently treated daily, either with vehicle or GSK503 for 35 consecutive days ( Fig. 5e,f ; Supplementary Fig. 5a ). This procedure reduced H3K27me3 levels in tumour and stromal cells without affecting Ezh2 levels, confirming inhibition of the catalytic function of Ezh2 ( Fig. 5g , Supplementary Fig. 5b ). Comparable to genetic ablation of Ezh2 , GSK503 treatment drastically reduced the emergence of new skin melanomas over time after treatment start ( Fig. 5h ; Supplementary Fig. 5c ). EZH2 is required for growth of human and murine melanoma Our findings demonstrate the requirement of Ezh2 for melanoma initiation. We hypothesized whether this might function through regulation of proliferation, since EZH2 has previously been associated with proliferation of human melanoma cells in vitro [28] , [29] , [30] . Interestingly, we observed a heterogeneity with respect to EZH2 expression in melanoma cells of both human biopsies as well as on Tyr::N-Ras Q61K Ink4a −/− skin tumours and metastases, ranging from high EZH2 expression to almost background levels ( Fig. 1a,b ; Supplementary Fig. 1 ). EZH2 highly expressing cells significantly correlated with KI67-positive cells, implicating EZH2-regulated proliferation of melanoma at primary tumour and metastatic sites ( Supplementary Fig. 6 ). To address the relevance of these findings for melanoma growth, we first blocked EZH2 activity in human melanoma cell cultures [43] , either by RNA interference-mediated silencing (RNAi) or by chemical inhibition using GSK503. In agreement with our in vivo findings, RNAi effectively reduced EZH2, while GSK503 application did not affect EZH2 levels. Both approaches, however, led to a considerable loss of H3K27me3 ( Supplementary Fig. 7a,b ). Notably, neither RNAi nor prolonged GSK503 application for 8 days did affect cell survival ( Supplementary Fig. 7c,d ). However, suppressing EZH2 activity stimulated a G1 cell cycle arrest ( Supplementary Fig. 7e,f ) and slowed down cell growth in culture ( Supplementary Fig. 7g,h ). To functionally study EZH2-regulated proliferation in vivo , we quantified proliferative cells in tumours of Tyr::N-Ras Q61K Ink4a −/− mice, either after Ezh2 cKO or GSK503 application ( Fig. 6a,c ). Both approaches led to a striking reduction of proliferative tumour cells ( Fig. 6b,d ). We next engrafted murine B16-F10 melanoma cells into C57Bl/6 mice ( Supplementary Fig. 8a ). Depletion of Ezh2 function using RNAi or GSK503 significantly reduced global H3K27me3 levels in vivo ( Supplementary Fig. 8b–e ). Importantly, EZH2 inactivation led to an inhibition of tumour growth ( Supplementary Fig. 8b,f ). Finally, we engrafted Tyr::N-Ras Q61K Ink4a −/− skin melanoma (RIM)-derived cells into athymic nude- Foxn1 nu/nu mice ( Fig. 6e ). These RIM allografts were confirmed to express various melanocytic markers, reassuring their melanoma origin ( Supplementary Fig. 8g,h ). RIMs were first allowed to reach a considerable size for 15 to 25 days after transplantation ( Fig. 6e,j ; Supplementary Fig. 8k,n ). Subsequent TM-induced Ezh2 cKO in growing RIMs completely abolished Ezh2 protein and H3K27me3, while GSK503 application significantly reduced H3K27me3 ( Fig. 6f–i ). This was associated with an inhibition of further tumour growth in both cKO and GSK503-treated samples ( Fig. 6f,j,k ; Supplementary Fig. 8i–n ), highlighting Ezh2 inactivation as an efficient strategy for blocking melanoma growth. 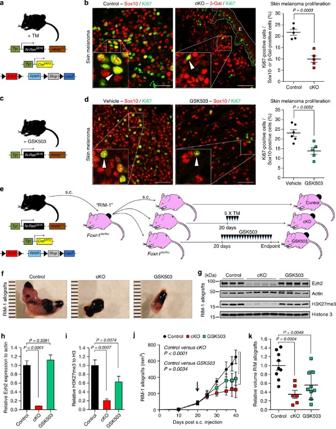Figure 6:Ezh2ablation and GSK503 treatment prevents murine melanoma growth. (a) Mouse genotypes and strategy as in (Fig. 5b) used to analyze the effect of conditionalEzh2ablation on melanoma proliferation inTyr::N-RasQ61KInk4a−/−mice. (b) Immunofluorescent staining on skin melanoma sections for Sox10 (control) or β-Gal (cKO) and Ki67 4 weeks after conditionalEzh2ablation to quantify a proliferation rate. White arrowheads, Sox10- or β-Gal-positive/Ki67-positive cells. (c) Mouse genotypes and strategy as in (Fig. 5f) used to analyze the effect of temporary GSK503 treatment on melanoma proliferation inTyr::N-RasQ61KInk4a−/−mice. (d) Immunofluorescent staining on skin melanoma sections for Sox10 and Ki67 4 weeks after treatment start with vehicle or GSK503 to quantify a proliferation rate. White arrowheads, Sox10-positive/Ki67-positive cells. (e) Mouse genotypes and strategy used to s.c. engraft and expandTyr::N-RasQ61KInk4a−/−mice-derived melanoma cells inFoxn1nu/nuanimals to analyze the effect of conditionalEzh2ablation and GSK503 treatment on melanoma growth. (f) Representative macroscopic pictures of control, cKO and GSK503-treated RIM-1 allografts. (g–i) Western blot for Ezh2 protein and H3K27me3 on lysed tumours from (f) to quantify loss of Ezh2 (h) and H3K27me3 (i). (j,k) Growth of control, cKO and GSK503-treated RIM-1 allografts (j) and relative tumour volume of all RIM allografts (j;Supplementary Fig. 8k,n) at endpoints (k). Black arrow, time point of TM application/start of GSK503 treatment. E, epidermis; s.c., subcutaneous. Data are represented as mean±s.e.m. ofn=5 (b), mean±s.e.m. ofn=6 (vehicle),n=5 (GSK503) (d), mean±s.e.m. ofn=3 (control),n=4 (cKO, GSK503) (g–j), mean±s.e.m. ofn=9 (control, GSK503),n=6 (cKO) (k).Pvalues calculated with unpaired Student’st-test (b,d), analysis of variance and Fisher’s least significant difference test (h–k). Scale bars, 50 μm (b,d), 1mm (f). Figure 6: Ezh2 ablation and GSK503 treatment prevents murine melanoma growth. ( a ) Mouse genotypes and strategy as in ( Fig. 5b ) used to analyze the effect of conditional Ezh2 ablation on melanoma proliferation in Tyr::N-Ras Q61K Ink4a −/− mice. ( b ) Immunofluorescent staining on skin melanoma sections for Sox10 (control) or β-Gal (cKO) and Ki67 4 weeks after conditional Ezh2 ablation to quantify a proliferation rate. White arrowheads, Sox10- or β-Gal-positive/Ki67-positive cells. ( c ) Mouse genotypes and strategy as in ( Fig. 5f ) used to analyze the effect of temporary GSK503 treatment on melanoma proliferation in Tyr::N-Ras Q61K Ink4a −/− mice. ( d ) Immunofluorescent staining on skin melanoma sections for Sox10 and Ki67 4 weeks after treatment start with vehicle or GSK503 to quantify a proliferation rate. White arrowheads, Sox10-positive/Ki67-positive cells. ( e ) Mouse genotypes and strategy used to s.c. engraft and expand Tyr::N-Ras Q61K Ink4a −/− mice-derived melanoma cells in Foxn1 nu/nu animals to analyze the effect of conditional Ezh2 ablation and GSK503 treatment on melanoma growth. ( f ) Representative macroscopic pictures of control, cKO and GSK503-treated RIM-1 allografts. ( g – i ) Western blot for Ezh2 protein and H3K27me3 on lysed tumours from ( f ) to quantify loss of Ezh2 ( h ) and H3K27me3 ( i ). ( j , k ) Growth of control, cKO and GSK503-treated RIM-1 allografts ( j ) and relative tumour volume of all RIM allografts ( j ; Supplementary Fig. 8k,n ) at endpoints ( k ). Black arrow, time point of TM application/start of GSK503 treatment. E, epidermis; s.c., subcutaneous. Data are represented as mean±s.e.m. of n =5 ( b ), mean±s.e.m. of n =6 (vehicle), n =5 (GSK503) ( d ), mean±s.e.m. of n =3 (control), n =4 (cKO, GSK503) ( g – j ), mean±s.e.m. of n =9 (control, GSK503), n =6 (cKO) ( k ). P values calculated with unpaired Student’s t -test ( b , d ), analysis of variance and Fisher’s least significant difference test ( h – k ). Scale bars, 50 μm ( b , d ), 1mm ( f ). Full size image EZH2 inactivation prevents metastatic spread of melanoma When depleting Ezh2 in our melanoma model before appearance of skin melanoma ( Supplementary Fig. 9a,b ), we observed that control mice, apart from skin tumours, frequently developed Sox10-positive melanoma metastases. However, conditional loss of Ezh2 almost fully prevented the generation of both lymph node and distant lung metastases, drastically increasing metastases-free survival ( Supplementary Fig. 9c–e ). Distant metastases likely arise from primary skin melanomas. Thus, a lack of metastases was expected, since early Ezh2 ablation also prevented emergence of skin tumours ( Fig. 4 ). To functionally analyze metastatic spread from cutaneous melanoma, we inactivated Ezh2 function in Tyr::N-Ras Q61K Ink4a −/− mice already bearing skin tumours ( Fig. 7a–c ). Strikingly, control animals consistently developed metastases, while Ezh2 cKO mice exhibited a significant reduction in melanoma-positive lymph nodes ( Fig. 7d ) and a virtual absence of distant metastases in the lung ( Fig. 7e ). Consequently, Ezh2 cKO mice displayed a highly increased melanoma-specific survival compared with controls ( Fig. 7f ). Likewise, GSK503-mediated Ezh2 inhibition counteracted formation of lymph node and lung metastases ( Fig. 7g,h ). Importantly, temporary inhibition of Ezh2 prolonged melanoma-specific survival compared with vehicle-treated animals, resulting in doubling of the median survival time ( Fig. 7i ). 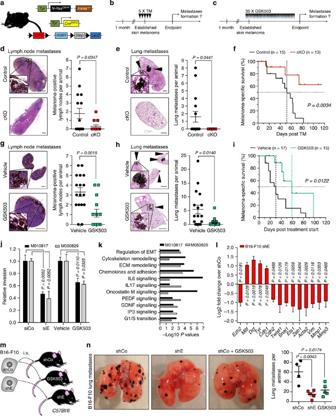Figure 7: EZH2 is required for metastatic progression of human and murine melanoma. (a–c) Mouse genotypes (a) and strategies (b,c) used to analyze the effect of conditionalEzh2ablation (b) and GSK503 treatment (c) on metastatic spread ofTyr::N-RasQ61KInk4a−/−skin melanoma. (d,e) Metastases count at day of sacrifice in lymph nodes (d) and lung (e) of control and cKO animals using macroscopic pictures, H&E staining and Sox10 staining on sections. Macroscopic pictures and Sox10 staining performed as in (Supplementary Fig. 9). Black arrowheads, lung metastases. (f) Kaplan–Meier curves comparing melanoma-specific survival after conditionalEzh2ablation. (g,h) Metastases count at day of sacrifice in lymph nodes (g) and lung (h) of vehicle- and GSK503-treated animals using macroscopic pictures, H&E staining and Sox10 staining on sections. Macroscopic pictures and Sox10 staining performed as in (Supplementary Fig. 9). Black arrowheads, lung metastases. (i) Kaplan–Meier curves comparing melanoma-specific survival during and after GSK503 treatment. (j) Quantification of relative invasive capacity of M010817 and M050829 following EZH2 depletion with siE or EZH2 inhibition using GSK503. (k) −Log10Pvalues based on gene ontology analysis using gene signatures of M010817 and M050829 after EZH2 depletion with siE (Supplementary Fig. 10). (l) Reverse transcription–qPCR for melanocyte and EMT genes on B16-F10 after Ezh2 depletion with shE. (m) Mouse genotypes and strategy used to i.v. engraft B16-F10 cells followingEzh2silencing using shE to analyze the effect of Ezh2 depletion and GSK503 treatment on metastases formation. (n) Representative macroscopic pictures of lungs from vehicle and GSK503-treated (from day 1 on until endpoint) animals to quantify lung metastases after i.v. engraftment of shCo and shE B16-F10 cells. ECM, extra cellular matrix; H&E, haematoxylin and eosin; i.v., intravenous. Data are represented as mean±s.e.m. ofn=15 (control)n=13 (cKO) (d,e), mean±s.e.m. ofn=17 (vehicle)n=15 (GSK503) (g,h), mean±s.e.m. ofn=4 (j), mean±s.e.m. ofn=3 (l), mean±s.e.m. ofn=4 (shCo)n=5 (shE, GSK503) (n).Pvalues calculated with unpaired Student’st-test (d,e,g,h,j), log-rank (Mantel–Cox) test (f,i), analysis of variance and Fisher’s least significant difference test (l,n). Scale bars, 500 μm (d,e), 1mm (g,h). Figure 7: EZH2 is required for metastatic progression of human and murine melanoma. ( a – c ) Mouse genotypes ( a ) and strategies ( b , c ) used to analyze the effect of conditional Ezh2 ablation ( b ) and GSK503 treatment ( c ) on metastatic spread of Tyr::N-Ras Q61K Ink4a −/− skin melanoma. ( d , e ) Metastases count at day of sacrifice in lymph nodes ( d ) and lung ( e ) of control and cKO animals using macroscopic pictures, H&E staining and Sox10 staining on sections. Macroscopic pictures and Sox10 staining performed as in ( Supplementary Fig. 9 ). Black arrowheads, lung metastases. ( f ) Kaplan–Meier curves comparing melanoma-specific survival after conditional Ezh2 ablation. ( g , h ) Metastases count at day of sacrifice in lymph nodes ( g ) and lung ( h ) of vehicle- and GSK503-treated animals using macroscopic pictures, H&E staining and Sox10 staining on sections. Macroscopic pictures and Sox10 staining performed as in ( Supplementary Fig. 9 ). Black arrowheads, lung metastases. ( i ) Kaplan–Meier curves comparing melanoma-specific survival during and after GSK503 treatment. ( j ) Quantification of relative invasive capacity of M010817 and M050829 following EZH2 depletion with siE or EZH2 inhibition using GSK503. ( k ) −Log10 P values based on gene ontology analysis using gene signatures of M010817 and M050829 after EZH2 depletion with siE ( Supplementary Fig. 10 ). ( l ) Reverse transcription–qPCR for melanocyte and EMT genes on B16-F10 after Ezh2 depletion with shE. ( m ) Mouse genotypes and strategy used to i.v. engraft B16-F10 cells following Ezh2 silencing using shE to analyze the effect of Ezh2 depletion and GSK503 treatment on metastases formation. ( n ) Representative macroscopic pictures of lungs from vehicle and GSK503-treated (from day 1 on until endpoint) animals to quantify lung metastases after i.v. engraftment of shCo and shE B16-F10 cells. ECM, extra cellular matrix; H&E, haematoxylin and eosin; i.v., intravenous. Data are represented as mean±s.e.m. of n =15 (control) n =13 (cKO) ( d , e ), mean±s.e.m. of n =17 (vehicle) n =15 (GSK503) ( g , h ), mean±s.e.m. of n =4 ( j ), mean±s.e.m. of n =3 ( l ), mean±s.e.m. of n =4 (shCo) n =5 (shE, GSK503) ( n ). P values calculated with unpaired Student’s t -test ( d , e , g , h , j ), log-rank (Mantel–Cox) test ( f , i ), analysis of variance and Fisher’s least significant difference test ( l , n ). Scale bars, 500 μm ( d , e ), 1mm ( g , h ). Full size image Metastatic spread of a human primary melanoma is usually initialized by gain of invasive capacity, which allows a cell to evade from the primary tumour site [44] . Accordingly, both RNAi and drug-mediated inhibition of EZH2 significantly reduced the invasive capacity of human melanoma cultures measured in a Boyden Chamber assay ( Fig. 7j ; Supplementary Fig. 9f ). Next, we used cell cultures derived from two distinct patients to perform a comparative global gene expression analysis of control versus EZH2-depleted melanoma cells ( Supplementary Fig. 10 ). Cluster analysis of transcriptionally regulated genes indicated that reducing EZH2 levels affected expression of genes involved, among others, in cytoskeleton remodelling, extra cellular matrix remodelling and EMT ( Fig. 7k ). In support of these findings, we observed a gain of melanocyte markers including microphthalmia-associated transcription factor (Mitf) and a loss of NCSC/EMT genes when depleting Ezh2 in murine B16-F10 melanoma cells ( Fig. 7l ). Notably, an increase in MITF has previously been connected to loss of invasive capacity [45] , while genes such as TWIST1 and ZEB1 are well-established drivers of NCSC delamination as much as of melanoma EMT and metastasis [6] , [46] . Finally, when inoculating B16-F10 cells intravenously into C57Bl/6 mice, RNAi and importantly also GSK503 treatment drastically reduced lung nodule counts ( Fig. 7m,n ). In summary, EZH2 is crucial throughout several steps of melanoma metastasis, such as EMT and homing to distant sites. Therefore, targeting Ezh2 in vivo efficiently prevented metastasis formation in our melanoma model, and pharmacological EZH2 inhibition might represent a promising treatment strategy in preventing metastasis in patients. EZH2 represses a set of genes connected to patient survival To further characterize the transcriptional programmes controlled by EZH2 activity in melanoma, based on the gene expression arrays ( Supplementary Fig. 10 ), we first defined genes significantly changed in both patient-derived cell cultures after EZH2 depletion ( Fig. 8a ). We next performed TCGA-based unbiased analyses to determine the clinical relevance of these EZH2-regulated genes. We correlated expression levels of each of these genes with disease outcome in patients using RNAseq and clinical data from TCGA. Strikingly, for 24% of all genes commonly upregulated upon EZH2 silencing, high expression levels in patients were associated with improved survival, while only 5.3% correlated with poor survival ( Fig. 8b ; Supplementary Table 2 ). Furthermore, for 19.6% of all genes commonly downregulated after EZH2 silencing, low expression levels in patients correlated with adverse survival ( Fig. 8c ). Thus, EZH2 activity predominantly suppresses a transcriptional programme beneficial for human patients and is associated with activation of a considerable fraction of genes linked to poor survival. 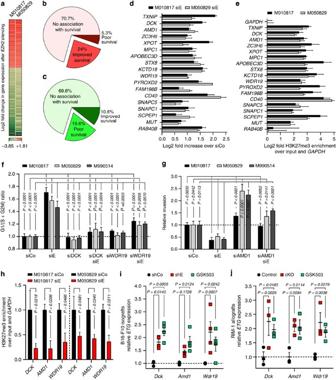Figure 8: EZH2 target genes are functionally involved in melanomagenesis. (a) Gene expression signature of M010817 and M050829 after EZH2 depletion using siE. Average log2 fold change values of three siE replicates compared with three siCo replicates in (Supplementary Fig. 10) and significantly changed in both cell lines are shown. (b,c) Summary of TCGA-based unbiased analyses of genes upregulated (b;Supplementary Table 2) or downregulated (c) in (a). For upregulated genes in (a), specimens with high RNAseq reads for the corresponding genes were compared with specimens with low RNAseq reads. For downregulated genes in (a), specimens with low RNAseq reads for the corresponding genes were compared with specimens with high RNAseq reads. (d) Reverse transcription–qPCR (RT–qPCR) for genes associated with improved survival in (b) on M010817 and M050829 after EZH2 depletion using siE (relative toGAPDH). (e) H3K27me3 ChIP and subsequent qPCR for promoters of genes associated with improved survival in (b) on untreated M010817 and M050829. (f) Quantification of G1/(S+G2M) ratio of M010817, M050829 and M990514 after depletion of EZH2 and DCK/WDR19 using siE and siDCK/siWDR19. (g) Quantification of relative invasive capacity of M010817, M050829 and M990514 after depletion of EZH2 and AMD1 using siE and siAMD1. (h) H3K27me3 ChIP and subsequent qPCR for gene promoters of selected ETGs on M010817 and M050829 after EZH2 depletion using siE. (i) RT–qPCR for selected ETGs on lysed shCo, shE and GSK503-treated B16-F10 tumours from (Supplementary Fig. 8b). (j) RT–qPCR for selected ETGs on lysed control, cKO and GSK503-treated RIM-1 tumours from (Fig. 6f). Data are represented as mean±s.e.m. ofn=3 (d,f–h,j), mean±s.e.m. ofn=4 (e), mean±s.e.m. ofn=3 (shCo),n=4 (shE, GSK503) (i).Pvalues calculated with analysis of variance and Fisher’s least significant difference test. Figure 8: EZH2 target genes are functionally involved in melanomagenesis. ( a ) Gene expression signature of M010817 and M050829 after EZH2 depletion using siE. Average log2 fold change values of three siE replicates compared with three siCo replicates in ( Supplementary Fig. 10 ) and significantly changed in both cell lines are shown. ( b , c ) Summary of TCGA-based unbiased analyses of genes upregulated ( b ; Supplementary Table 2 ) or downregulated ( c ) in ( a ). For upregulated genes in ( a ), specimens with high RNAseq reads for the corresponding genes were compared with specimens with low RNAseq reads. For downregulated genes in ( a ), specimens with low RNAseq reads for the corresponding genes were compared with specimens with high RNAseq reads. ( d ) Reverse transcription–qPCR (RT–qPCR) for genes associated with improved survival in ( b ) on M010817 and M050829 after EZH2 depletion using siE (relative to GAPDH ). ( e ) H3K27me3 ChIP and subsequent qPCR for promoters of genes associated with improved survival in ( b ) on untreated M010817 and M050829. ( f ) Quantification of G1/(S+G2M) ratio of M010817, M050829 and M990514 after depletion of EZH2 and DCK/WDR19 using siE and siDCK/siWDR19. ( g ) Quantification of relative invasive capacity of M010817, M050829 and M990514 after depletion of EZH2 and AMD1 using siE and siAMD1. ( h ) H3K27me3 ChIP and subsequent qPCR for gene promoters of selected ETGs on M010817 and M050829 after EZH2 depletion using siE. ( i ) RT–qPCR for selected ETGs on lysed shCo, shE and GSK503-treated B16-F10 tumours from ( Supplementary Fig. 8b ). ( j ) RT–qPCR for selected ETGs on lysed control, cKO and GSK503-treated RIM-1 tumours from ( Fig. 6f ). Data are represented as mean±s.e.m. of n =3 ( d , f – h , j ), mean±s.e.m. of n =4 ( e ), mean±s.e.m. of n =3 (shCo), n =4 (shE, GSK503) ( i ). P values calculated with analysis of variance and Fisher’s least significant difference test. Full size image The genes upregulated upon EZH2 silencing and associated with improved patient survival were, first, confirmed to be transcriptionally elevated after EZH2 depletion in human melanoma cell cultures. Indeed, messenger RNA of all 18 genes (24% in Fig. 8b ) was significantly increased after EZH2 depletion ( Fig. 8d ; Supplementary Table 3 ). Second, chromatin immunoprecipitation (ChIP) assays for H3K27me3 were performed to determine whether these 18 genes are direct targets of EZH2-mediated histone methylation. Intriguingly, 17 out of these 18 analyzed genes exhibited promoter regions highly enriched for H3K27me3 in comparison to GAPDH promoter as negative control, indicating that these genes are targets of EZH2-dependent transcriptional repression ( Fig. 8e ; Supplementary Table 3 ). EZH2 targets are functionally distinct suppressors of melanoma To relate these EZH2 target genes (ETG) functionally to aspects of melanomagenesis, we performed functional screens in human melanoma cell cultures. We focussed on a potential rescue of, first, EZH2 depletion-induced G1 cell cycle arrest and, second, EZH2 depletion-induced loss of invasive capacity. Among the tested ETGs, deoxycytidine kinase ( DCK ), adenosylmethionine decarboxylase 1 (AMD1) and WD repeat domain 19 ( WDR19 ) displayed promising features. We first established efficient RNAi-mediated silencing of these ETGs ( Supplementary Fig. 11a ). ETG silencing did not affect the efficiency of EZH2 knockdown achieved by siEZH2 ( Supplementary Fig. 11b ). However, EZH2 silencing-dependent upregulation of DCK , AMD1 or WDR19 was strongly counteracted with the double RNAi approach ( Supplementary Fig. 11c ). Interestingly, when simultaneously depleting EZH2 and DCK or WDR19, the G1 cell cycle arrest induced by EZH2 silencing was significantly reverted ( Fig. 8f ; Supplementary Fig. 11d,f ). Depletion of AMD1, however, was not sufficient to induce such a rescue ( Supplementary Fig. 11d ). In contrary, simultaneous depletion of EZH2 and AMD1 efficiently led to a regain of the invasive capacity that was lost upon silencing of EZH2 alone ( Fig. 8g ; Supplementary Fig. 11e,g ). DCK and WDR19 silencing, however, had no effect on invasion of human melanoma cells ( Supplementary Fig. 11e ). We then reconfirmed these genes as direct ETGs through a ChIP assay on control and EZH2-depleted cells. Indeed, upon RNAi targeting of EZH2 , H3K27me3 mark was significantly reduced in promoter regions of DCK , AMD1 and WDR19 loci ( Fig. 8h ). Importantly, in both B16-F10 isografts and RIM-1 allografts ( Fig. 6f ; Supplementary Fig. 8b ) Dck , Amd1 and Wdr19 were consistently upregulated upon Ezh2 inactivation through either cKO (or RNAi) or GSK503 treatment ( Fig. 8i,j ), identifying these ETGs as likely tumour suppressors in vivo . Thus, throughout melanomagenesis, EZH2 might dynamically repress diverse tumour suppressor genes to achieve either favourable growth or invasion kinetics. AMD1 suppresses EMT and metastatic spread of melanoma Interestingly, silencing of AMD1 in human melanoma cultures induced an increase in invasion on its own ( Fig. 8g ; Supplementary Fig. 11e,g ). Therefore, we further focused on the relevance of this tumour suppressor in preventing melanoma EMT and metastasis. Based on TCGA, patients with low AMD1 expression displayed a significantly shorter overall survival as compared with those with high AMD1 expression ( Fig. 9a ). Further, stage I–III patients of the AMD1 low group showed a considerably reduced distant metastases-free survival ( Fig. 9b ). Comparably, low AMD1 expression correlated with more advanced vertical invasion of primary melanomas ( Fig. 9c ). Finally, depletion of AMD1 in human melanoma cells induced expression of NCSC/EMT-relevant genes including SNAI1 , TWIST1 and ZEB1 ( Fig. 9d ). Similarly, when silencing Amd1 in B16-F1 ( Supplementary Fig. 11h ), a murine melanoma cell line with negligible metastatic potential, a comparable EMT gene set was upregulated ( Fig. 9e ). Therefore, to functionally link loss of Amd1 to metastasis, we first intravenously transplanted Amd1 -silenced B16-F1 cells into C57Bl/6 mice ( Fig. 9f ). Strikingly, loss of Amd1 strongly induced nodule formation in the lung ( Fig. 9g ). Next, we depleted Amd1 in highly metastatic B16-F10 cells ( Supplementary Fig. 11i ). Comparable to B16-F1, Amd1 silencing further enhanced the metastatic potential of B16-F10 cells. Most importantly, when inhibiting lung nodule formation through Ezh2 inactivation by GSK503 treatment, depletion of Amd1 was sufficient to significantly re-induce metastasis ( Fig. 9h ). Thus, during melanomagenesis EZH2 epigenetically represses the tumour suppressor AMD1 allowing metastatic spread, while EZH2-targeted therapy successfully counteracts disease progression. 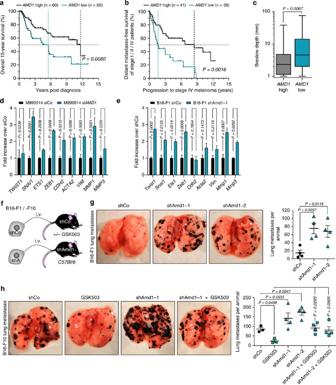Figure 9:The EZH2 target geneAMD1is a tumour suppressor that prevents melanoma metastasis. (a) Kaplan–Meier curves comparing overall survival of melanoma specimens (stage I–IV) with respect toAMD1transcript levels based on TCGA. (b) Kaplan–Meier curves comparing distant metastases-free survival of stage I–III melanoma specimens (primary melanoma/lymph node metastases) with respect toAMD1transcript levels based on TCGA. (c) Breslow depths of melanoma specimens’ primary melanomas with respect toAMD1transcript levels based on TCGA. (d) Reverse transcription–qPCR (RT–qPCR) for EMT genes on M990514 after AMD1 depletion with siAMD1. (e) RT–qPCR for EMT genes on B16-F1 after Amd1 depletion with shAmd1. (f) Mouse genotypes and strategies used to i.v. engraft B16-F1/B16-F10 cells followingAmd1silencing using shAmd1 to analyze the effect of Amd1 depletion and GSK503 treatment on metastases formation. (g) Representative macroscopic pictures of lungs fromC57Bl/6animals after i.v. engraftment of shCo and shAmd1 B16-F1 cells to quantify lung metastases. (h) Representative macroscopic pictures of lungs from vehicle and GSK503-treated (from day 1 on until endpoint) animals to quantify lung metastases after i.v. engraftment of shCo and shAmd1 B16-F10 cells.AMD1low/high, bottom and top 60 patients with respect toAMD1transcript levels; i.v., intravenous; shA, shAmd1. Data are represented as median±100% range ofn=48 (AMD1high),n=43 (AMD1low) (c), mean±s.e.m. ofn=3 (d,e), mean±s.e.m. ofn=4 (g,h),n=3 (shCo, GSK503 inh).Pvalues calculated with log-rank (Mantel–Cox) test (a,b), unpaired Student’st-test (c), analysis of variance and Fisher’s least significant difference test (d,e,g,h). Figure 9: The EZH2 target gene AMD1 is a tumour suppressor that prevents melanoma metastasis. ( a ) Kaplan–Meier curves comparing overall survival of melanoma specimens (stage I–IV) with respect to AMD1 transcript levels based on TCGA. ( b ) Kaplan–Meier curves comparing distant metastases-free survival of stage I–III melanoma specimens (primary melanoma/lymph node metastases) with respect to AMD1 transcript levels based on TCGA. ( c ) Breslow depths of melanoma specimens’ primary melanomas with respect to AMD1 transcript levels based on TCGA. ( d ) Reverse transcription–qPCR (RT–qPCR) for EMT genes on M990514 after AMD1 depletion with siAMD1. ( e ) RT–qPCR for EMT genes on B16-F1 after Amd1 depletion with shAmd1. ( f ) Mouse genotypes and strategies used to i.v. engraft B16-F1/B16-F10 cells following Amd1 silencing using shAmd1 to analyze the effect of Amd1 depletion and GSK503 treatment on metastases formation. ( g ) Representative macroscopic pictures of lungs from C57Bl/6 animals after i.v. engraftment of shCo and shAmd1 B16-F1 cells to quantify lung metastases. ( h ) Representative macroscopic pictures of lungs from vehicle and GSK503-treated (from day 1 on until endpoint) animals to quantify lung metastases after i.v. engraftment of shCo and shAmd1 B16-F10 cells. AMD1 low/high, bottom and top 60 patients with respect to AMD1 transcript levels; i.v., intravenous; shA, shAmd1. Data are represented as median±100% range of n =48 ( AMD1 high), n =43 ( AMD1 low) ( c ), mean±s.e.m. of n =3 ( d , e ), mean±s.e.m. of n =4 ( g , h ), n =3 (shCo, GSK503 in h ). P values calculated with log-rank (Mantel–Cox) test ( a , b ), unpaired Student’s t -test ( c ), analysis of variance and Fisher’s least significant difference test ( d , e , g , h ). Full size image In this study, we demonstrate EZH2 to be a key player in promoting malignant melanoma progression in a genetic mouse model of cutaneous melanoma. Importantly, conditional deletion of Ezh2 did not interfere with normal melanocyte function and benign dermal hyperplasia, underlining the particular roles of EZH2 in melanoma growth and progression to metastatic disease. In support of this, temporary pharmacological inhibition of Ezh2 counteracted growth and metastasis in vivo , and blocking EZH2 activity in human melanoma cells affected their growth as well as invasive capacity. In line with these findings, human melanoma patients showed particularly poor survival when EZH2 transcript levels were high or when a newly identified set of EZH2 target genes was expressed at low levels. Importantly, these target genes displayed tumour-suppressive functions affecting either melanoma growth or metastatic spread. Hence, EZH2 activity exhibits two functionally distinct roles in driving malignant melanoma progression that appear to be highly relevant for human patients. In many tissues as much as in corresponding malignancies a central function of EZH2 is to sustain stem cell identity and proliferation by transcriptional repression of senescence and differentiation genes [17] , [22] . For instance, in normal and cancerous breast epithelial cells, EZH2 induces stemness features, while in vivo Ezh2 expression initializes hyperplasia in mammary glands [25] , [26] . In haematopoietic stem cells, Ezh2 prevents exhaustion of the stem cell pool in aged mice [20] , and Ezh2 function is also essential for maturation of early B-cell progenitors and for B-cell germinal centre formation [27] , [47] , [48] . Activating Ezh2 Y646N mutations induce B-cell germinal centre hyperplasia resulting in lymphoma [27] , while in a model of acute myeloid leukaemia, Ezh2 is required for leukemogenicity [49] . In contrast, in NCSCs, the embryonic progenitors of melanocytes, Ezh2 regulates the acquisition of a mesenchymal fate rather than stem cell maintenance [21] . Similarly, in certain epithelial tumours EZH2 has been associated with EMT and cellular migration, rather than tumour cell growth [50] , [51] . Therefore, to elucidate the role of Ezh2 in a given cell type, the proper cellular and physiological context has to be considered. For melanoma, this is best achieved in transgenic mice, in which melanoma is initiated and spontaneously grows in an undisturbed environment without prior ex vivo manipulation of tumour cells [52] . Indeed, the function of EZH2 in selected melanoma cell lines has been controversial and linked to control of proliferation or in vitro migration [28] , [29] , [30] . Taking advantage of an inducible and cKO strategy that allows functional gene investigation at different stages of disease in an intact environment, we show that Ezh2 plays a dual role during melanomagenesis. Ezh2 is required for malignant tumour growth at initial stages of melanoma formation, but a striking effect of Ezh2 inactivation is also on metastatic spread of melanoma. The process of melanoma metastasis is thought to be triggered by acquisition of mesenchymal features [44] . Thus, the role of Ezh2 in melanoma in vivo appears to be analogous, at least in part, to its function in embryonic neural crest development. A few previous in vivo studies have also taken advantage of the cKO technique in genetic mouse models of melanoma, although most reports on gene function in melanoma are based on cell culture and xenotransplantation assays. However, up to date, genes shown to be involved in melanoma formation turned out to be also important for normal melanocytes and benign hyperplasia cells [14] , [31] , [41] , [53] . In contrast, Ezh2 plays a unique tumour-specific role in melanoma and is not required for normal melanocyte function, in accordance with the strong upregulation of its expression during malignant melanoma progression. Thus, unlike in many other cancers and their tissues of origin, EZH2 function appears to be of no relevance for the cells from which melanoma arises from. Based on TCGA and two further datasets [9] , [38] , cutaneous melanoma is the only solid cancer with recurring EZH2 Y646* gain-of-function mutations. It will be of interest to investigate whether EZH2 WT and especially EZH2 Y646* operate as de novo oncogenic drivers of metastasizing melanoma. Since EZH2 acts as a transcriptional repressor [17] , genes upregulated on EZH2 silencing are likely candidates for being direct targets of EZH2-mediated H3K27me3. In agreement with this, promoters of genes selected based on our TCGA analyses were indeed confirmed to be enriched in H3K27me3. Of note, these selected ETGs are not only potential indicators of improved patient survival, but have also been linked to characteristics relevant for tumour progression. For instance, loss of DCK was correlated with resistance to cytarabine and decitabine treatments of different cancers [54] . AMD1 , another gene upregulated upon EZH2 silencing, is involved in the biosynthesis of the non-canonical amino acid hypusine, and has recently been identified as part of a metabolic tumour suppressor network in lymphoma [55] , [56] . Finally, WDR19 is a component of the intraflagellar transport machinery and has been associated with good prognosis in prostate cancer [57] , [58] . While epigenetic repression of DCK and WDR19 supported melanoma cell growth, repression of AMD1 induced EMT and metastasis of melanoma cells. Interestingly, alterations in biosynthesis networks, such as amino acid and nucleotide metabolism, have recently been demonstrated to be essential for EMT and metastasis [59] . Likewise, EZH2-mediated repression of AMD1-linked hypusine biosynthesis might thus contribute to EMT and metastatic spread of cutaneous melanoma. In the future, an unbiased screen for further EZH2-target genes might provide additional candidate factors possibly involved in melanoma disease progression. Dependent on the mutational landscape, levels of oxidative and metabolic stress and the stromal context, the set of aberrantly silenced tumour suppressor genes might be assembled differently in a given melanoma and at a given time point. However, EZH2 itself represents a central node in the control of melanoma progression through epigenetic regulation of such genes. In support of this, pharmacological inhibition of Ezh2 using the preclinical drug GSK503 in melanoma-bearing mice efficiently counteracted metastatic melanoma progression, resulting in a doubled survival time. Further, GSK503 also prevented metastasis formation of transplanted melanoma cells through, at least partly, Amd1 de-repression. Melanoma patients die of metastatic disease and not of primary tumour growth [1] . Therefore, novel therapeutic strategies effectively interfering with metastatic spread are required. Recently, several chromatin-modifying drugs have been successfully applied in preclinical cancer models and are likely to be taken forward to clinical trials [60] . Accordingly, our study reveals that EZH2 inhibition might be a promising strategy for future therapies of human melanoma patients. Human biopsies Human biopsies were isolated and genotyped as described [43] . Usage of naevus and melanoma biopsies as well as melanoma-derived cell cultures was approved by the official ethical authorities of Canton of Zurich, Switzerland. Written informed consent was obtained from all subjects and approved by the local institutional review boards (EK647 and EK800). Mice Tyr::N- Ras Q61K animals and Ink4a -defficient mice have previously been described [14] , [34] , [61] . The Tyr::Cre ERT2 line [14] , [31] , [39] , Ezh2 lox animals [19] , [21] and R26R::LacZ mice [40] have been analyzed elsewhere. Mouse genotyping was performed according to a standard DNA isolation protocol [62] , followed by PCR using a Taq PCR Core Kit (201225, Qiagen) and primers indicated in ( Supplementary Table 4 ). Genetic background of ( Tyr::N-Ras Q61K Ink4a −/− ) Tyr::Cre ERT2 Ezh2 lox/lox R26R::LacZ mice was mixed, while background of Tyr::N-Ras Q61K Ink4a −/− animals was Black 6. Mice were born with the expected ratio of Mendelian inheritance, and no changes in gender ratios were observed. Transgenic mice used were of both genders and were subjected to experiments either at the age of 1 month or on tumour development (5 to 7 months). Melanoma-developing mice were frequently monitored and killed at an endpoint defined by adverse clinical symptoms, such as multiple skin tumours (Ø>5 mm), weight loss (Δ m >15%) or hunched back. Three-month-old female C57Bl/6J and athymic nude- Foxn1 nu/nu mice were purchased (Charles River Laboratories). Mice engrafted subcutaneously with melanoma cells were killed at an endpoint defined by tumour volume ( V >1,000 mm 3 ). Tumour volume was calculated as follows: V =2/3 × π × (( a + b )/4)) 3 , where a (mm) was the length and b (mm) was the width of the tumour. Mice engrafted intravenously with melanoma cells were killed 12 days post engraftment. All animal experiments have been approved by the veterinary authorities of Canton of Zurich, Switzerland, and were performed in accordance with Swiss law and the GlaxoSmithKline policy on the Care, Welfare and Treatment of Animals. In vivo TM and GSK503 application To conditionally ablate Ezh2 , ( Tyr::N-Ras Q61K Ink4a −/− ) Tyr::Cre ERT2 Ezh2 lox/lox R26R::LacZ mice were subjected to treatment with TM (T5648, Sigma-Aldrich), which was diluted (10 mg ml −1 ) in ethanol and sunflower oil (1:9). Conditional ablation of Ezh2 was achieved by daily intraperitoneal injections of 2 mg TM for 5 consecutive days. Mice were either 4 weeks old or at an age of 5 to 7 months, when first skin melanomas had become macroscopically detectable (Ø≥2 mm). To pharmacologically inhibit Ezh2 activity, Tyr::N-Ras Q61K Ink4a −/− , Ink4a −/− and C57Bl/6 mice were subjected to treatment with GSK503 (ref. 27 ), which was diluted (15 mg ml −1 ) in 20% Captisol solution (Cydex). Efficient Ezh2 inhibition was achieved by daily intraperitoneal injections of 150 mg kg −1 GSK503 over 35 consecutive days. Ink4a −/− and C57Bl/6 mice were 5 months old. Tyr::N-Ras Q61K Ink4a −/− animals were at an age of 5 to 7 months, when first skin melanomas had become macroscopically detectable (Ø≥2 mm). Mice were monitored during and after treatment to measure GSK503-induced reversible weight loss. Moreover, a few GSK503-treated animals developed ascites, independently of the genotype, and had to be excluded from the studies. C57Bl/6 and Foxn1 nu/nu mice engrafted with melanoma cells were subjected to TM and GSK503 treatment as described above. Quantification of skin melanomas and metastases When Ezh2 ablation was done at 1 month, developing trunk skin lesions were considered as melanomas above a diameter of 2 mm (Ø≥2 mm). At day of sacrifice, a final skin melanoma count was established. In cKO mice, whole mount X-Gal staining was used to quantify recombined tumours and X-Gal-negative tumours were excluded from cKO melanoma count. To quantify metastases, accessory axillary, proper axillary, sciatic and subiliac lymph nodes (total of eight) as well as the lungs were subjected to further analyses. Lymph nodes were considered melanoma positive, when Sox10-positive cells were found on histological sections. Black dots on lung surface were counted and confirmed as melanoma metastases using Sox10 staining on histological sections. Melanoma-specific survival curves were based on presence of (recombined) skin melanomas and/or metastases. When Ezh2 ablation or GSK503 treatment was done in established melanoma, newly forming skin melanomas (Ø≥2 mm) were counted weekly. At day of sacrifice, skin melanoma and metastases counts were established as described for early Ezh2 ablation, except skin melanoma numbers were not based on recombination but solely on tumour numbers. Melanoma-specific survival curves were based on the presence of newly formed skin melanomas and/or metastases. Isografting and allografting of murine melanoma cells Skin melanomas from Tyr::N-Ras Q61K Ink4a −/− ( Tyr::Cre ERT2 Ezh2 lox/lox R26R::LacZ ) animals were dissociated into small pieces using forceps and scissors. Tissue was digested using 0.25 mg ml −1 Liberase DH Research Grade (05401054001, Roche) in RPMI 1640 (42401, Life Technologies) for 45 min at 37 °C followed by a treatment with 0.55 mg ml −1 Dispase II (17105, Life Technologies) and 0.2 mg ml −1 DNase I (10104159001, Roche) for 15 min at 37 °C. Single cells were separated from remaining tissue using a 70 μm cell strainer and engrafted subcutaneously into Foxn1 nu/nu mice in PBS or cultured in vitro using growth medium as described below. Foxn1 nu/nu mice were subcutaneously engrafted with either 500,000 RIM-1 cells, 500,000 RIM-2 cells or 1 Mio RIM-3 cells. C57Bl/6 mice were either subcutaneously engrafted with 1 Mio B16-F10 cells or tail vein injected with 400,000 B16-F1 cells/100,000 B16-F10 cells. Histological analysis and immunofluorescence Human and mouse tissue samples were fixed in 4% buffered formaldehyde and embedded in paraffin, except for whole mount X-Gal staining. Therefore, mouse tissue samples were fixed in formaldehyde for 20 min and subjected to X-Gal staining as described [14] . Human samples were processed into sections of 3 μm thickness, while mouse samples were processed into 5 μm sections. Slides were stained with haematoxylin and eosin according to standard protocols. Sections were subjected either to immunohistochemical analyses or to immunofluorescent analyses. Briefly, immunohistochemical stainings were performed using primary antibodies ( Supplementary Table 5 ) in combination with the iVIEW DAB Detection Kit (760-091, Ventana) or the ChemMate Detection Kit (K5006, Dako) according to manufacturers’ protocols. For immunofluorescence, protocols described elsewhere were applied [14] . Briefly, sections were deparaffinized and subjected to an antigen retrieval step using citrate buffer (S2369, Dako). Primary antibodies ( Supplementary Table 5 ) were applied in blocking buffer (1% BSA in PBS and 0.05% Triton X-100) overnight at 4 °C and visualized using secondary antibodies ( Supplementary Table 6 ) in blocking buffer for 1 h at room temperature. For visualization of β-Gal, a biotin α-chicken (1:300, AP194B, Merck Millipore) secondary antibody was combined with further signal amplification using horse radish peroxidase–streptavidin (1:300, 016-030-084, Jackson ImmunoResearch) and the TSA Plus Cy3 Kit (1:50, NEL744001KT, PerkinElmer) according to manufacturers’ protocol. Subsequently, nuclei were stained with Hoechst 33342 (14533, Sigma-Aldrich) and slides were mounted with Fluorescent Mounting Medium (S3023, Dako). Immunohistochemical/fluorescent sections were analyzed using either a Mirax Midi Slide Scanner (Zeiss) or a DMI 6000B microscope (Leica). EZH2 mutagenesis and mutation analysis EZH2 mutations were chosen based on specimens in the Somatic Mutations data set for skin cutaneous melanoma as described below. Specimens showing non-synonymous mutations in the coding sequence of EZH2 and for which clinical data was available were selected. A previously validated pRetro-X construct containing human EZH2 WT , EZH2 Y646N or EZH2 Y646F complementary DNA (cDNA) was used [27] . Further mutations were introduced into EZH2 WT cDNA using a QuikChange II Site-Directed Mutagenesis Kit (200523, Agilent Technologies) according to manufacturer’s protocol. For each mutation, 10 ng of template EZH2 WT cDNA was used with the appropriate primers containing the corresponding sequence modification ( Supplementary Table 7 ), and constructs were sequenced using three pairs of primers covering the EZH2 sequence ( Supplementary Table 8 ). Cell cultures Human melanoma cell cultures were characterized before [43] , XB2 and Melan-a cell lines were previously described [63] , and HEK293T, B16-F1 and B16-F10 cell lines were purchased (ATCC). All cells (including primary RIM cells) were cultured in growth medium, which was RPMI 1640 supplemented with 10% FCS (16140, Life Technologies), 4 mM L-Glutamine (25030, Life Technologies), penicillin–streptomycin (15070, Life Technologies) and Fungizone Antimycotic (15290, Life Technologies) as previously specified [14] , [43] . Cell transfections and GSK503 treatment To overexpress EZH2 WT and mutated EZH2 , HEK293T cells were grown in growth medium devoid of antibiotics and transfected with 10 μg EZH2 -expressing plasmids using 2.5 M CaCl 2 in HEPES buffer according to standard protocols, and cells were subjected to functional analyses after 36 h. To temporarily deplete EZH2, DCK, AMD1 and WDR19, human melanoma cells were transfected with small interfering RNAs (siRNA) indicated in ( Supplementary Table 9 ). siRNA (25 nM) was applied in combination with jetPRIME siRNA Transfection Reagent (114-15, Polyplus Transfection) according to manufacturer’s guidelines. Growth medium was exchanged after 24 h and cells were subjected to further assays after 72 h, unless specified. For all functional assays the most efficient siRNAs underlined in ( Supplementary Table 9 ) were used. To stably deplete Ezh2 and Amd1, murine melanoma cells were transfected with small hairpin RNA-expressing plasmids indicated in ( Supplementary Table 9 ). Plasmid (10 μg) was applied in combination with jetPEI DNA Transfection Reagent (101-10 N, Polyplus Transfection) according to manufacturer’s guidelines. Transfected cells were selected using 1 μg ml −1 puromycin (A11138-02, Life Technologies) for 1 week before subjection to further assays. Efficiency of shEzh2 was previously validated [51] . To pharmacologically inhibit EZH2, melanoma cells were treated either with vehicle (DMSO) or 1 μM GSK503. Cells were treated for 8 days before subjection to further assays. Drug was only replenished when cells were passaged during the 8-day period. Cell growth and apoptosis assays To establish growth curves, cell counts were measured daily starting 48 h after transfection. For cell cycle analysis, cells were 50% ethanol fixed and labelled with propidium iodide including RNase A (F10797, Life Technologies). To measure apoptosis, an Annexin V Apoptosis Detection Kit (559763, BD Biosciences) was used. Cell cycle and apoptotic cells were quantified using a BD FACSCanto II flow cytometer (BD Biosciences) and FlowJo software (Tree Star). Boyden chamber invasion assay After 24 h of transfection or 8 days of GSK503 treatment, cells were starved for 48 h in starvation medium containing all supplements except 1% FCS. Subsequent Boyden Chamber invasion assays were done according to manufacturer’s protocol. Briefly, 150,000 cells were subjected to matrigel-coated well inserts (354480, BD Biosciences) in empty medium (0% FCS and 0% L-Glutamine). Growth medium was used as chemoattractant for 24 h. Transvaded cells were 4% buffered formaldehyde fixed and visualized using Hoechst 33342. Membranes were mounted to glass slides, and cell numbers were quantified using a DMI 6000B microscope and CellProfiler software [64] . Immunofluorescence on cells Cells were grown on cover slips, 50% ethanol fixed and subjected to immunofluorescent labelling using primary antibodies ( Supplementary Table 5 ) in blocking buffer (1% BSA in PBS) overnight at 4 °C and secondary antibodies ( Supplementary Table 6 ) for 1 h at room temperature. Nuclei were stained with Hoechst 33342, and cells were recorded with a DMI 6000B microscope. Protein isolation and Western blotting Protein isolation and Western blotting was done as previously described [14] , unless specified. Briefly, cells were lysed in RIPA buffer (89900, Thermo Scientific) containing Halt Phosphatase and Protease Inhibitor Cocktail (78420, 87786, Thermo Scientific), while tumour biopsies were homogenized in such buffer using a tissue homogeniser (Polytron). SDS–PAGE was carried out on 4–20% Mini-PROTEAN TGX Gels (456–1094, Bio Rad). Primary antibodies ( Supplementary Table 5 ) were applied in Odyssey blocking buffer (927–40000, LI-COR Biosciences) overnight at 4 °C and visualized using secondary antibodies ( Supplementary Table 6 ) in Odyssey blocking buffer for 45 min at room temperature. Blots were scanned and quantified with an Odyssey imaging system (LI-COR Biosciences). Quantified band intensities were normalized using either β-Actin or H3 as housekeeping protein. Full scans are shown in ( Supplementary Fig. 12 ). RNA isolation and reverse transcription–qPCR RNA extraction and DNase treatment of samples was performed using the RNeasy Mini Kit (74104, Qiagen) and the RNase-Free DNase Set (79254, Qiagen) according to manufacturer’s guidelines. Purified RNA was quantified using nanodrop and subjected to reverse transcriptase reaction using Maxima First Strand cDNA Synthesis Kit (K1641, Thermo Scientific) followed by an RNase H (EN0202, Thermo Scientific) digestion step according to manufacturer’s recommendations. Real-time quantitative PCR (qPCR) was performed on a LightCycler 480 System (Roche) using LightCycler 480 SYBR Green I Master (4707516001, Roche). Primers used are indicated in ( Supplementary Tables 10 and 11 ). Each sample was analyzed in technical triplicates, and relative quantified RNA was normalized using USF1 or GAPDH , when specified, as housekeeping transcript. Chromatin isolation and ChIP Chromatin isolation and ChIP was done as previously described [65] . Briefly, an antibody against H3K27me3 (1:250, 9733, Cell Signaling Technology) and Dynabeads Protein A (10002D, Life Technologies) were used. Real-time qPCR was performed on a Rotor Gene RG-3000 A (Qiagen) using the SensiFAST Probe Hi-ROX Kit (BIO-82005, Bioline). Primers were designed to amplify genomic DNA from a region flanking the transcriptional starting site −500 bp to +100 bp devoid of local CpG islands using CpG island prediction [66] . Primers used are indicated in ( Supplementary Table 12 ). Relative promoter enrichment was normalized to chromatin inputs and to GAPDH promoter as negative control. Microarray analysis Total RNA was isolated as described for reverse transcription–qPCR. Total RNA was amplified and biotin labelled using the MessageAmp II-Biotin Enhanced aRNA Amplification Kit (AM1791, Life Technologies). Biotin-labelled RNA was hybridized to Human Gene 2.1 ST Array (902136, Affymetrix) following the manufacturer’s protocol. After hybridization, microarrays were washed and stained using a GeneChip Fluidics Station 450 (Affymetrix) and scanned with a GeneChip Scanner 7G (Affymetrix). Differential gene expression was determined by R package limma [67] . Gene ontology network analysis was performed with MetaCore (Thomson Reuters). TCGA analysis The RNAseq, somatic mutations and clinical data sets for skin cutaneous melanoma and the somatic mutations data sets for colon adenocarcinoma, lung squamous cell carcinoma, lung adenocarcinoma, glioblastoma multiforme, kidney renal clear cell carcinoma, acute myeloid leukaemia, head and neck squamous cell carcinoma, breast invasive carcinoma and prostate adenocarcinoma were downloaded on 29 September 2013 from TCGA ( http://cancergenome.nih.gov/ ). Somatic mutation data was annotated using ANNOVAR [68] . Non-synonymous EZH2 mutations were mapped to functional EZH2 domains based on previous reports [17] , [18] . Raw RNAseq reads were normalized with edgeR [69] and differential RNA expression was analyzed with voom from R package limma [67] . Specimens with top and bottom transcript levels for a gene of interest were used for analysis. Patient numbers were gradually increased from a minimum of top and bottom 7% (19 out of 274) to a maximum of top and bottom 25% (69 out of 274) to optimize potential segregation of Kaplan–Meier curves. This procedure was performed for EZH2 and all commonly differentially expressed genes form the microarray data sets ( Fig. 8a ) in an unbiased way. Statistical analyses Quantifications of immunofluorescent stainings were done on sections of at least three different mice. Therefore, at least 150 hair follicles or at least 300 label-positive cells were counted. Cell culture-based experiments were done at least in biological triplicates. P values for comparison of two groups were calculated with unpaired Student’s t -test, except for paired data (follow-up measurements on the same mouse). Therefore, paired Student’s t -test was applied. P values for comparison of multiple groups were calculated with analysis of variance and Fisher’s least significant difference test. P values for comparison of Kaplan–Meier curves were calculated with log-rank (Mantel–Cox) test. P<0.05 was considered significant. How to cite this article: Zingg, D. et al . The epigenetic modifier EZH2 controls melanoma growth and metastasis through silencing of distinct tumour suppressors. Nat. Commun. 6:6051 doi: 10.1038/ncomms7051 (2015). Accession codes. Microarray data have been deposited in the NCBI Gene Expression Omnibus (GEO) archive under the accession code GSE63165 .